Normal muscle regeneration requires tight control of muscle cell fusion by tetraspanins CD9 and CD81 Skeletal muscle regeneration after injury follows a remarkable sequence of synchronized events. However, the mechanisms regulating the typical organization of the regenerating muscle at different stages remain largely unknown. Here we show that muscle regeneration in mice lacking either CD9 or CD81 is abnormal and characterized by the formation of discrete giant dystrophic myofibres, which form more quickly in the absence of both tetraspanins. We also show that, in myoblasts, these two tetraspanins associate with the immunoglobulin domain molecule CD9P-1 (EWI-F/FPRP), and that grafting of CD9P-1-depleted myoblasts in regenerating muscles also leads to abnormal regeneration. In vitro myotubes lacking CD9P-1 or both CD9 and CD81 fuse with a higher frequency than normal myotubes. Our study unveils a mechanism preventing inappropriate fusion of myotubes that has an important role in the restitution of normal muscle architecture during muscle regeneration. The skeletal muscle has a remarkable capacity to regenerate after mechanical or pathological injury. Muscle regeneration occurs in two main phases: the initial degenerative phase is characterized by necrosis of the damaged tissue and activation of an inflammatory response [1] . In the repair phase, the necrotic debris is phagocytosed, and regeneration of myofibres occurs for a large part through the action of satellite cells, skeletal muscle adult stem cells that are located beneath the muscle fibre basal lamina. Primarily quiescent, they can activate on injury and either self-renew or proliferate and further differentiate to become fusion-competent myoblasts [2] , [3] . Then, according to the severity of the myotrauma, these differentiated myoblasts fuse together to form new multinucleated myofibres or fuse to damaged myofibres. Once fusion of myogenic cells is completed, newly formed myofibres increase in size and under normal conditions, the regenerated muscle is morphologically and functionally indistinguishable from undamaged muscle, strongly suggesting that this process is tightly regulated. However, the regulatory mechanisms that allow the proper reconstitution of muscle architecture remain largely unknown. A crucial step during the regeneration process is the fusion of myoblasts. Studies in Drosophila and in the mouse have yielded considerable molecular information about the proteins mediating the attraction, adhesion and fusion of myoblasts [4] , [5] . These studies have in particular highlighted the key role of several intracellular proteins, many of them involved in the regulation of cytoskeleton dynamics and have identified a number of surface proteins required for recognition and adhesion of myoblasts but without any intrinsic fusogenic property [4] , [5] . Some of the molecules which are important for optimal myoblast fusion in vitro , including myoferlin [6] , Mannose receptor [7] , Fak [8] , PKCθ (ref. 9 ), have been demonstrated to be necessary for normal muscle regeneration in the mouse. In general, their absence yields delayed or abnormal regeneration characterized with properly aligned myofibres, but of reduced diameter, consistent with a decreased number of fusion events. Besides myoblast fusion, physiological cell–cell fusion in mammals occurs in three circumstances: between the egg and the sperm during fertilization, during the differentiation of macrophages into osteoclasts and giant cells, and for the formation of syncytiotrophoblast during placenta formation [10] . In pathological conditions, cell–cell fusion is induced by a number of viruses, including HIV, and is also a frequent property of tumour cells [11] . Among the molecules that have been shown to have a role in several cell–cell fusion events are the tetraspanins CD9 and CD81. Indeed, the ability of CD9 −/− oocytes to fuse with sperm is severely impaired [12] . CD81 −/− mice are hypofertile and CD9 −/− ::CD81 −/− mice are completely infertile, suggesting a cooperative role of CD9 and CD81 in sperm/egg fusion [13] . However, both CD9 and CD81 negatively regulate HIV-induced cell fusion [14] and macrophage fusion [15] . Altogether, these studies indicate that CD9 and CD81 can act both as positive and negative regulators of cell–cell fusion processes. A major characteristic of tetraspanins is their ability to interact with one another and many other surface proteins, thus building a dynamic network of interactions referred to as the ‘tetraspanin web’. Through this ‘web’, tetraspanins are believed to have a role in membrane compartmentalization [16] , [17] , [18] . This network follows a hierarchical, multi-step assembly process with specific tetraspanins associating in a first step with specific non-tetraspanin partners via direct protein–protein interaction. In a second step, these dimeric complexes can associate with one another via lipid-mediated tetraspanin–tetraspanin interactions. CD9 and CD81 share two common molecular partners, CD9P-1 (also known as EWI-F or FPRP) and EWI-2 (PGRL/IgSF8), members of the Immunoglobulin Superfamily [19] , [20] , [21] , [22] . Very few studies have addressed the function of these two molecules: EWI-2 expression was shown to modulate integrin functions [23] , [24] , and the ability of CD81 to support Plasmodium and hepatitis C virus infection of hepatocytic cells is reduced by CD9P-1 (ref. 25 ) and a truncated form of EWI-2 (ref. 26 ), respectively. The role of CD9 and CD81 in myogenesis and muscle regeneration has not been thoroughly investigated. CD9 and CD81 monoclonal antibodies were shown to slightly delay the formation of myotubes by the C2C12 muscle cells, and to trigger apoptotic degeneration of C2C12 myotubes in vitro [27] . In addition, ectopic expression of CD9 in a rhabdomyosarcoma cell line increased syncytia formation [27] . In the present study, we show that the absence of CD9 and CD81 yields abnormal muscle regeneration in vivo and a hyperfusion phenotype in vitro , due to a large extent to the fusion between myotubes. We also show that these two tetraspanins associate with CD9P-1 in primary myoblasts, and that depletion of this protein by RNA-mediated interference recapitulates the phenotype produced by the absence of CD9 and CD81. Our data reveal a molecular mechanism involving CD9, CD81 and CD9P-1 that prevents the fusion of myotubes and have an essential role in the control of skeletal muscle architecture during muscle regeneration. Upregulation of CD9 and CD81 in regenerating skeletal muscles Immunostaining of tibialis anterior (TA) muscle sections from C57BL/6 mice revealed that both tetraspanins are expressed in the muscle ( Fig. 1a and Supplementary Fig. S1a ). Colabelling with CD31 indicated that CD9 and CD81 are mainly expressed by endothelial cells of endomysial capillaries ( Supplementary Fig. S1b ). However, myofibres expressed a low level of CD81 ( Supplementary Fig. S1b , arrow head) but no detectable CD9. Importantly, using muscle sections from Tg:Pax7-nGFP mice (the paired/homeodomain transcription factor Pax7 is a marker of all satellite cells [28] ), we observed that satellite cells expressed both CD9 and CD81 ( Supplementary Fig. S1c,d ). 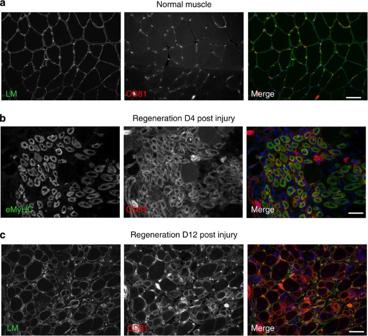Figure 1: Expression of CD81 in normal and regenerating adult skeletal muscle. Cryosections of mouse tibialis anterior (TA) were stained with antibodies to CD81 (red) and Laminin (LM) or embryonic myosin heavy chain (eMyHC) in green, as indicated and analysed by fluorescence microscopy. (a) Expression of CD81 in normal muscle; (b) 4 days post notexin injection CD81 is upregulated in activated myoblasts as judged by its coexpression with eMyHC. (c) Twelve days post notexin injection CD81 is strongly expressed in regenerating fibres (see alsoSupplementary Figs S1 and S2). For all images the scale bar is 50 μm. Figure 1: Expression of CD81 in normal and regenerating adult skeletal muscle. Cryosections of mouse tibialis anterior (TA) were stained with antibodies to CD81 (red) and Laminin (LM) or embryonic myosin heavy chain (eMyHC) in green, as indicated and analysed by fluorescence microscopy. ( a ) Expression of CD81 in normal muscle; ( b ) 4 days post notexin injection CD81 is upregulated in activated myoblasts as judged by its coexpression with eMyHC. ( c ) Twelve days post notexin injection CD81 is strongly expressed in regenerating fibres (see also Supplementary Figs S1 and S2 ). For all images the scale bar is 50 μm. Full size image To examine the expression of CD9 and CD81 in regenerating muscle, when fusion occurs, we first used the mouse model of notexin-induced acute myoinjury. Four days after injury, the regenerating muscle is characterized by the presence of numerous nascent myofibres, which strongly expressed CD81 as shown by the colabelling with an anti-embryonic myosin antibody ( Fig. 1b ). CD9 is highly expressed by inflammatory cells recruited in the damaged tissue but remained undetectable on these nascent myofibres ( Supplementary Fig. S2a ). Both CD81 ( Fig. 1c ) and CD9 ( Supplementary Fig. S2b ) were expressed by centrally nucleated myofibres formed 12 days after myoinjury, and their expression levels strongly decreased 4 weeks after injury, a time point characterized by ad integrum restitution of the tissue ( Supplementary Fig. S2c ). We also studied the expression of both tetraspanins in the Mdx4cv mouse, a model for Duchenne muscular dystrophy presenting a complete lack of dystrophin [29] . These mice represent a model of chronic muscle regeneration, and are characterized by foci of muscle degeneration/regeneration. This model confirmed the upregulation of CD81 in nascent myofibres and of CD9 at later stages of regeneration ( Supplementary Fig. S2d,e ). Expression of CD9 and CD81 in mouse primary myoblasts To further characterize the expression of CD9 and CD81 in myogenic cells, we isolated mouse satellite cells and examined the expression of these two tetraspanins in proliferating and differentiating primary myoblasts. Western blot ( Fig. 2a ) and flow cytometry ( Fig. 2b ) showed that both tetraspanins are expressed in undifferentiated myoblasts and that their expression levels increase on differentiation concomitantly with differentiation markers such as myosin or troponin ( Fig. 2a ) to reach a maximal expression level after 2 or 3 days. Confocal microscopy indicated that CD81 ( Fig. 2c ), and to a lesser extent CD9 (data not shown), colocalized with M-cadherin, which has been shown to have a role in myoblast fusion in vitro , at sites of myoblast–myotube or myotube–myotube contacts ( Fig. 2c , arrow). In addition, the labelling of CD81 revealed the existence of short and parallel M-cadherin-negative filopodium-like protrusions between myotubes, not yet described to our knowledge ( Fig. 2d ). CD81 was also localized at the tips of myotubes ( Fig. 2e ), which make frequent contacts with neighbouring muscle cells ( Fig. 2f ). 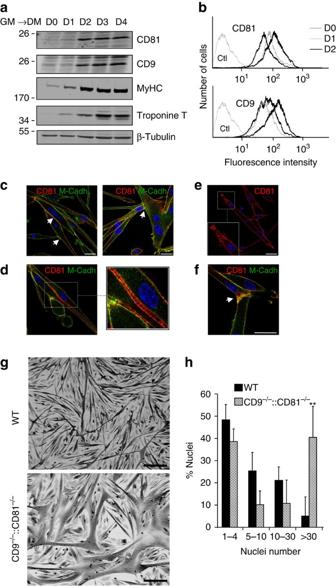Figure 2: CD9 and CD81 are expressed in mouse primary myoblasts and regulate fusionin vitro. The expression of CD9 and CD81 was studied in primary cultures of myoblasts induced to undergo differentiation. (a) By western blot, the expression levels of CD9 and CD81 increase concomitantly with differentiation markers such as myosin or troponin. (b) Flow cytometry analysis shows that CD9 and CD81 are expressed at the surface of undifferentiated myoblasts and that their expression levels increase after induction of differentiation (Ctl: nonspecific fluorescence). (c) Two examples of CD81 localization in differentiated myoblasts as determined by fluorescence confocal microscopy: CD81 (red) partially colocalizes with M-cadherin (M-Cadh, green), in myoblast/myotubes and myotube/myotube contact areas (arrow). (d) CD81 staining reveals short and parallel filopodium-like protrusions between myotubes (higher magnification is shown on the right). (e) CD81 is enriched at myotubes tips, which make frequent contacts with neighbouring muscle cells (arrow) (f). Scale bar inc–fis 25 μm. (g) Myoblasts isolated from 8-week-old littermate control and CD9/CD81 null mice were plated at equal density and induced to differentiate. After 3 days of differentiation, cells were fixed and stained with May Grundwald Giemsa. Representative microscopic fields are presented. Scale bar, 200 μm. (h) Ten fields of each condition were photographed at × 10 magnification and nuclei were counted. The histogram shows the mean±s.d. of the percentage of nuclei in cells with different numbers of nuclei and is representative of at least three different experiments (**P<0.01 compared with the control sample, Mann–Whitney test). Figure 2: CD9 and CD81 are expressed in mouse primary myoblasts and regulate fusion in vitro . The expression of CD9 and CD81 was studied in primary cultures of myoblasts induced to undergo differentiation. ( a ) By western blot, the expression levels of CD9 and CD81 increase concomitantly with differentiation markers such as myosin or troponin. ( b ) Flow cytometry analysis shows that CD9 and CD81 are expressed at the surface of undifferentiated myoblasts and that their expression levels increase after induction of differentiation (Ctl: nonspecific fluorescence). ( c ) Two examples of CD81 localization in differentiated myoblasts as determined by fluorescence confocal microscopy: CD81 (red) partially colocalizes with M-cadherin (M-Cadh, green), in myoblast/myotubes and myotube/myotube contact areas (arrow). ( d ) CD81 staining reveals short and parallel filopodium-like protrusions between myotubes (higher magnification is shown on the right). ( e ) CD81 is enriched at myotubes tips, which make frequent contacts with neighbouring muscle cells (arrow) ( f ). Scale bar in c – f is 25 μm. ( g ) Myoblasts isolated from 8-week-old littermate control and CD9/CD81 null mice were plated at equal density and induced to differentiate. After 3 days of differentiation, cells were fixed and stained with May Grundwald Giemsa. Representative microscopic fields are presented. Scale bar, 200 μm. ( h ) Ten fields of each condition were photographed at × 10 magnification and nuclei were counted. The histogram shows the mean±s.d. of the percentage of nuclei in cells with different numbers of nuclei and is representative of at least three different experiments (** P <0.01 compared with the control sample, Mann–Whitney test). Full size image CD9 and CD81 negatively regulate muscle cell fusion in vitro To get further insights into the role of CD9 and CD81 in myoblast fusion, primary myoblasts from mutant and wild-type (WT) mice were analysed for their ability to differentiate in culture. Myoblasts from CD9 −/− or CD81 −/− mice generated myotubes that were very similar to those produced by WT myoblasts (data not shown). In contrast, CD9 −/− ::CD81 −/− myoblasts generated large syncytia that contained more than 30 nuclei ( Fig. 2g ). Several independent isolates of CD9 −/− ::CD81 −/− myoblasts displayed similar characteristics. Altogether, these data indicate that CD9 and CD81 cooperate to negatively regulate myoblast fusion in vitro . CD9P-1 and EWI-2 associate with CD9 and CD81 in myoblasts The function of tetraspanins is tightly linked to the transmembrane proteins they associate with [16] . We therefore looked for CD9 and CD81 molecular partners that could have a role in myoblast fusion. The major biotin-labelled surface proteins coimmunoprecipitated with CD9 and CD81 comigrated with CD9P-1 and EWI-2, both in proliferating and differentiated myoblasts ( Fig. 3a ). The coimmunoprecipitation of these two molecules with CD9 and CD81 was confirmed by western blot ( Fig. 3b ). Reciprocally, both anti-CD9P-1 and anti-EWI-2 antibodies coimmunoprecipitated a fraction of both tetraspanins ( Fig. 3b ). These data demonstrate that CD9P-1 and EWI-2 associate with CD9 and CD81 at the surface of primary myoblasts. Moreover, as observed with CD9 and CD81, the surface expression level of CD9P-1 increased in myoblasts after 2 days in differentiation medium as determined by flow cytometry ( Fig. 3c ). In addition, CD9P-1 is weakly expressed on normal muscle ( Supplementary Fig. S3a ) and during the regeneration process its expression increased in muscle cells where it colocalized with CD81 ( Supplementary Fig. S3b ). 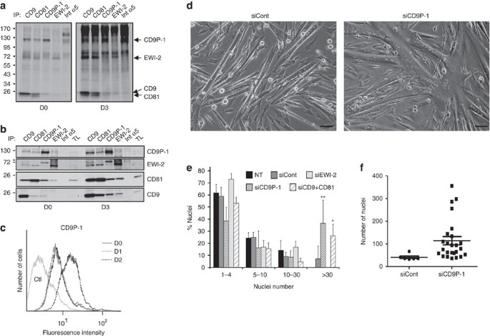Figure 3: CD9P-1 associates with CD9 and CD81 and negatively regulates myoblast fusion. (a) After biotinylation of cell surface proteins, proliferating myoblasts (D0) or after 3 days in differentiation medium (D3) were lysed with Brij97 and immunoprecipitations (IP) were performed as indicated on the top of each lane. The proteins in the immunoprecipitates were revealed using IRdye800-conjugated streptavidin. Bands corresponding to CD9P-1, EWI-2, CD81 and CD9 are indicated on the right. Note that the integrin β1 subunit comigrates with CD9P-1. Inb, the composition of the different IPs was analysed by Western blot. As a control, an anti-integrin α5 (Int. α5) antibody did not coimmunoprecipitate CD9, CD81 or CD9P-1. TL, total cell lysate. Asterisk (*) indicates a nonspecific band. (c) Flow cytometry analysis shows that CD9P-1 is expressed at the surface of undifferentiated myoblasts and its expression increases after 2 days in differentiation conditions (Ctl: nonspecific fluorescence). (d) Primary myoblasts were transfected with a siRNA oligonucleotide targeting CD9P-1 (siCD9P-1) or with a control siRNA (siCont); contrast phase: representative microscopic fields after 48 h of differentiation. Scale bar, 50 μm. (e) Primary myoblasts were left untransfected (NT) or were transfected with a siRNA oligonucleotide targeting CD9P-1 (siCD9P-1), EWI-2 (siEWI-2), both CD9 and CD81 (siCD9+CD81) or with a control siRNA (siCont). After 48 h of differentiation, cells were fixed and ten fields of each condition were photographed at × 10 magnification and nuclei were counted. The histogram shows the mean±s.d. of the percentage of nuclei in cells with different numbers of nuclei and is representative of at least three different experiments. Ø: not observed. (f) Number of nuclei in control or CD9P-1-silenced myotubes containing more than 30 nuclei. Note that this quantification underestimates the number of nuclei in the largest syncitia because only the part of the syncitium observed in each field is taken into consideration (**P<0.01, *P<0.05 as compared with the control, Mann–Whitney test). Figure 3: CD9P-1 associates with CD9 and CD81 and negatively regulates myoblast fusion. ( a ) After biotinylation of cell surface proteins, proliferating myoblasts (D0) or after 3 days in differentiation medium (D3) were lysed with Brij97 and immunoprecipitations (IP) were performed as indicated on the top of each lane. The proteins in the immunoprecipitates were revealed using IRdye800-conjugated streptavidin. Bands corresponding to CD9P-1, EWI-2, CD81 and CD9 are indicated on the right. Note that the integrin β1 subunit comigrates with CD9P-1. In b , the composition of the different IPs was analysed by Western blot. As a control, an anti-integrin α5 (Int. α5) antibody did not coimmunoprecipitate CD9, CD81 or CD9P-1. TL, total cell lysate. Asterisk (*) indicates a nonspecific band. ( c ) Flow cytometry analysis shows that CD9P-1 is expressed at the surface of undifferentiated myoblasts and its expression increases after 2 days in differentiation conditions (Ctl: nonspecific fluorescence). ( d ) Primary myoblasts were transfected with a siRNA oligonucleotide targeting CD9P-1 (siCD9P-1) or with a control siRNA (siCont); contrast phase: representative microscopic fields after 48 h of differentiation. Scale bar, 50 μm. ( e ) Primary myoblasts were left untransfected (NT) or were transfected with a siRNA oligonucleotide targeting CD9P-1 (siCD9P-1), EWI-2 (siEWI-2), both CD9 and CD81 (siCD9+CD81) or with a control siRNA (siCont). After 48 h of differentiation, cells were fixed and ten fields of each condition were photographed at × 10 magnification and nuclei were counted. The histogram shows the mean±s.d. of the percentage of nuclei in cells with different numbers of nuclei and is representative of at least three different experiments. Ø: not observed. ( f ) Number of nuclei in control or CD9P-1-silenced myotubes containing more than 30 nuclei. Note that this quantification underestimates the number of nuclei in the largest syncitia because only the part of the syncitium observed in each field is taken into consideration (** P <0.01, * P <0.05 as compared with the control, Mann–Whitney test). Full size image CD9P-1 negatively regulates muscle cell fusion in vitro To investigate the potential role of CD9P-1 and EWI-2 in myoblast fusion, we analysed the differentiation of primary myoblasts after silencing these molecules by RNA-mediated interference ( Fig. 3 and Supplementary Fig. S4 ). CD9P-1-silenced myoblasts formed large syncytia, which could contain several hundreds of nuclei ( Fig. 3d–f ). These large syncitia could be observed after 2 or 3 days in differentiation medium, while it took 3 or 4 days for CD9 −/− ::CD81 −/− myoblasts to generate similar syncytia. Similar results were obtained with two different short interfering RNA (siRNA) oligonucleotides, ruling out possible off-target effects ( Supplementary Fig. S4c ). The silencing of EWI-2 did not change myoblast fusion ( Fig. 3e ). Double silencing of CD9 and CD81 also induced the formation of large syncytia ( Fig. 3e ), confirming the phenotype obtained with myoblasts from CD9 −/− ::CD81 −/− mice. Of note, CD9P-1 silencing was efficient and did not modify the expression levels of CD9 and CD81 ( Supplementary Fig. S4a,b ). Lack of CD9P-1 or CD9 and CD81 promotes myotube fusion To further understand how the lack of CD9P-1 could induce the formation of large syncytia, we analysed by time-lapse videomicroscopy the behaviour of cells treated with a control siRNA or a siRNA targeting CD9P-1 during the differentiation process ( Fig. 4 and Supplementary Movies 1 and 2 ). The first hours of differentiation are characterized by elongation and migration of myoblasts, which were similar in both conditions. After 24 h, only few cells had fused. At this stage, there was a twofold increase in the number of multinucleated cells after depletion of CD9P-1 (9±0.4% versus 4±1.4%; about 1,000 cells examined). Moreover, 1.4% of CD9P-1-depleted cells had already 5−10 nuclei (versus 0 for control cells). Thus, the absence of CD9P-1 leads to an increase of the fusion of myoblasts. 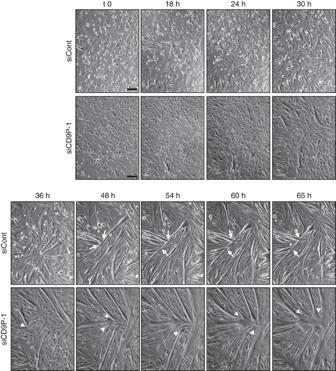Figure 4: Lack of CD9P-1 promotes the fusion of myotubes. Primary myoblasts were transfected with a control siRNA (siCont) or with a siRNA oligonucleotide targeting CD9P-1 (siCD9P-1) and recorded by time-lapse videomicroscopy. Images were acquired at 10-min intervals. The arrow shows a contact between two WT myotubes that is not followed by fusion and the arrowheads show the fusion between CD9P-1-depleted myotubes. Scale bars, 100 μm. See alsoSupplementary Movies 1and2. Figure 4: Lack of CD9P-1 promotes the fusion of myotubes. Primary myoblasts were transfected with a control siRNA (siCont) or with a siRNA oligonucleotide targeting CD9P-1 (siCD9P-1) and recorded by time-lapse videomicroscopy. Images were acquired at 10-min intervals. The arrow shows a contact between two WT myotubes that is not followed by fusion and the arrowheads show the fusion between CD9P-1-depleted myotubes. Scale bars, 100 μm. See also Supplementary Movies 1 and 2 . Full size image The myotubes formed in both conditions were very mobile and their tips highly dynamic, allowing frequent contacts between myotubes. Despite these contacts, control myotubes in particular the large ones rarely fused with one another. In contrast, after depletion of CD9P-1 many large myotubes fused with one another with a high efficiency: most myotubes fused at least once with other myotubes during the course of the recording, and many myotubes underwent several successive fusions with neighbouring myotubes leading to the formation of giant branched syncytia ( Fig. 4 , 48–65 h and Supplementary Movies 1 and 2 ). Similarly, we observed that the branched structures formed by CD9 −/− ::CD81 −/− myoblasts also resulted from the fusion of myotubes ( Supplementary Movie 3 ). From these data we conclude that the increased size of the syncytia observed in the absence of CD9P-1 or both CD9 and CD81 is due not only to an increase in the rate of myoblast fusion, but also and mainly to a dramatic increase in the number of myotubes fusing with each other. Dystrophic muscle regeneration in the absence of CD9 or CD81 Finally, we investigated whether the hyperfusion phenotype observed in the absence of CD9 and CD81 in vitro was associated with a defect of regeneration ( Fig. 5 ). Uninjured tibialis anterior muscles of CD9 −/− , CD81 −/− and CD9 −/− ::CD81 −/− mice were morphologically normal ( Fig. 5a–d ). Four days after notexin injury, WT regenerating muscles displayed myoblasts/nascent myofibres containing 2 or 3 centrally located nuclei and an eosinophilic cytoplasm. At this time point, there was no major difference in CD9 −/− or CD81 −/− mice compared with the control mice, except for the presence of some nascent myofibres containing more than three nuclei ( Fig. 5f ). Twelve days after notexin injection, control muscles contained numerous centronucleated myofibres with a diameter of 34.5±9.11 μm. The regenerating muscles of CD9 −/− or CD81 −/− mice showed several abnormalities: the myofibres had an increased diameter (57.5±11.2 and 69.4±12 μm, respectively) associated with a greater size distribution (15–98 μm in mutant mice versus 18–54 μm in control mice). In addition, many of the myofibres were dystrophic ( Fig. 5i–k ): they were hyperchromatic, eosinophilic (an hallmark of high cytoplasmic protein content) and contained numerous elongated nuclei. Both the cytoplasmic compartment and nuclei formed whorls frequently separated by vacuoles. Importantly, the regeneration defect is accelerated in CD9 −/− ::CD81 −/− mice. Indeed, the regenerating muscles of these mice displayed, 4 days after notexin injection, numerous hyperchromatic multinucleated myoblasts, some of which containing centrally located chains of nuclei ( Fig. 5h ). Moreover, at this stage, we already observed some giant dystrophic myofibres ( Fig. 5h ), similar to those observed only 12 days post injury in single knockout mice. Finally, the muscles of mutant animals failed to restore a normal architecture 1 month after notexin injection, in contrast to the muscles of control animals. In particular, many dystrophic structures were still observed at this stage ( Fig. 5n–p ). 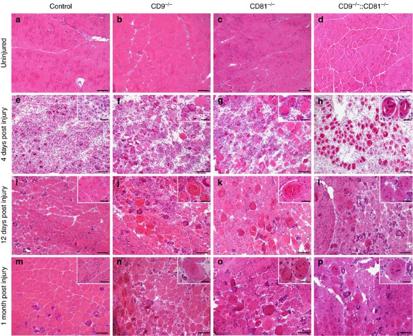Figure 5: Muscle regeneration is abnormal in the absence of CD9 or CD81. Representative cross-sections of control, CD9−/−, CD81−/−and CD9−/−::CD81−/−TA stained with haematoxylin and eosin. (a–d) Uninjured; (e–h) 4 days after notexin injection; (i–l) 12 days after notexin injection; (m–p) 1 month after notexin injection. Examples of normal or dystrophic structures are shown at higher magnification in inset. Scale bars, 100 μm; insets, 50 μm. Figure 5: Muscle regeneration is abnormal in the absence of CD9 or CD81. Representative cross-sections of control, CD9 −/− , CD81 −/− and CD9 −/− ::CD81 −/− TA stained with haematoxylin and eosin. ( a – d ) Uninjured; ( e – h ) 4 days after notexin injection; ( i – l ) 12 days after notexin injection; ( m – p ) 1 month after notexin injection. Examples of normal or dystrophic structures are shown at higher magnification in inset. Scale bars, 100 μm; insets, 50 μm. Full size image Analysis of longitudinal sections confirmed the formation of abnormal myofibres during the regeneration process in the absence of CD9 and/or CD81. Twelve days post injury, the regenerating fibres of control mice had a diameter <60 μm and a single chain of centrally located nuclei ( Fig. 6a ). Mutant mice showed regenerating myofibres of diameters >100 μm, some of which containing several parallel chains of nuclei ( Fig. 6c–f ). In addition, some of these large myofibres were in the continuity of two myofibres of normal size ( Fig. 6d–f (arrow)). These morphological features are compatible with the fusion of two myofibres. 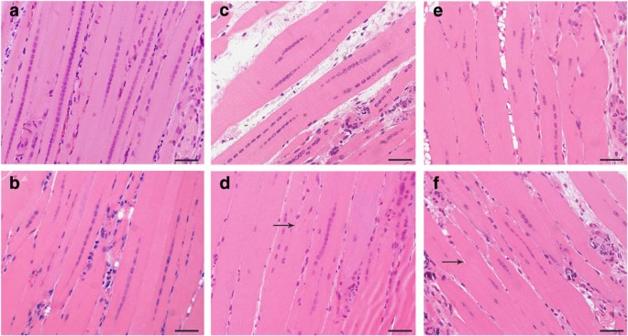Figure 6: Longitudinal sections of regenerating muscles from normal and CD9/CD81 mutant mice. Haematoxylin and eosin staining of 1 μm resin-embedded longitudinal sections of regenerating muscles 12 days after notexin injection. (a,b) Normal control mice showing classical features of regenerating fibres forming fibres with centrally located nuclei. (c–f) Mutant mice showing large regenerating myofibres, many of which containing several parallel chains of nuclei. Arrows indicate the apparent merging of two myofibres. (c) CD81−/−mutant, (d) CD9−/−::CD81−/−mutant, (e,f) CD9−/−mutant. Scale bar, 50 μm. Figure 6: Longitudinal sections of regenerating muscles from normal and CD9/CD81 mutant mice. Haematoxylin and eosin staining of 1 μm resin-embedded longitudinal sections of regenerating muscles 12 days after notexin injection. ( a , b ) Normal control mice showing classical features of regenerating fibres forming fibres with centrally located nuclei. ( c – f ) Mutant mice showing large regenerating myofibres, many of which containing several parallel chains of nuclei. Arrows indicate the apparent merging of two myofibres. ( c ) CD81 −/− mutant, ( d ) CD9 −/− ::CD81 −/− mutant, ( e , f ) CD9 −/− mutant. Scale bar, 50 μm. Full size image To further characterize the dystrophic structures of CD9 −/− ::CD81 −/− animals, transverse sections were stained for laminin, actin bundles (using phalloidin) or α-actinin (a z-disc component [30] ; Fig. 7 ). In WT sections, actin staining displayed a granular aspect, consistent with a transversal sectioning of parallel myofibrils ( Fig. 7a ). In many dystrophic structures of mutant animals, this granular aspect coexisted with a staining of actin bundles in different orientations ( Fig. 7b ). The occurrence in some dystrophic structures of areas displaying a punctuated α-actinin staining pattern, adjacent to regions showing a striated staining pattern, was also coherent with the presence in the same myofibres of myofibrils in different orientations ( Fig. 7e and Supplementary Fig. S5 ). Moreover, the α-actinin labelling revealed another feature of the dystrophic myofibres. While in WT transversal muscle sections, due to the alignment of z-discs, the α-actinin labelling in each individual myofibre is in the same plane, in dystrophic myofibres of mutant animals the uneven z-planes staining of α-actinin revealed contiguous areas in which z-discs were not aligned ( Fig. 7b ). This misalignment of z-discs was particularly apparent for ring-like structures, in which the periphery and the central part of the structure have misaligned myofibrils ( Fig. 7f ). Some of these structures contained discontinuous internal laminin and compressed nuclei at the junction of the two parts of the structure ( Fig. 7c and Supplementary Fig. S5 ). 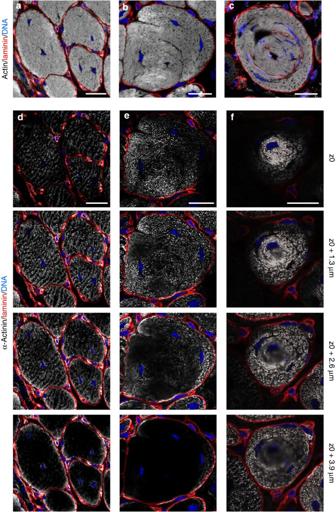Figure 7: Actin and α-actinin organizations in regenerating myofibres. Fluorescence confocal microscopy analyses of cryosections of TA from control and mutants mice 12 days after notexin injection. (a–c) Three-dimensional projections from 1.3 μm z-stack of sections stained with 4',6-diamidino-2-phenylindole (DAPI; blue), an anti-laminin antibody (red) and phalloidin (grey) to reveal actin (a: control mice;b: CD9−/−::CD81−/−;c: CD9−/−). (d–f) Three-dimensional projections from successive 1.3 μm z-stack of cryosections stained with DAPI (blue), an anti-laminin antibody (red) and an anti-α-actinin antibody (grey) (d: control mice;e: CD9−/−::CD81−/−;f: CD81−/−). Note that the same sections are analysed inaandd, as well as inbande. For all images the scale bar is 20 μm. See alsoSupplementary Fig. S4. Figure 7: Actin and α-actinin organizations in regenerating myofibres. Fluorescence confocal microscopy analyses of cryosections of TA from control and mutants mice 12 days after notexin injection. ( a – c ) Three-dimensional projections from 1.3 μm z-stack of sections stained with 4',6-diamidino-2-phenylindole (DAPI; blue), an anti-laminin antibody (red) and phalloidin (grey) to reveal actin ( a : control mice; b : CD9 −/− ::CD81 −/− ; c : CD9 −/− ). ( d – f ) Three-dimensional projections from successive 1.3 μm z-stack of cryosections stained with DAPI (blue), an anti-laminin antibody (red) and an anti-α-actinin antibody (grey) ( d : control mice; e : CD9 −/− ::CD81 −/− ; f : CD81 −/− ). Note that the same sections are analysed in a and d , as well as in b and e . For all images the scale bar is 20 μm. See also Supplementary Fig. S4 . Full size image Absence of CD9P-1 in myoblast alters muscle regeneration Finally, to determine whether the lack of CD9P-1 also affects regeneration in vivo , we grafted control and CD9P-1-silenced myoblasts into regenerating TA muscles 24 h after a cardiotoxin injury. As early as 4 days post-grafting, the engraftment of CD9P-1-silenced cells, in contrast to control cells, yielded the formation of the typical giant dystrophic myofibres ( Fig. 8 ) observed in the absence of CD9 or CD81. These aberrant structures were also characterized by a disorganization of the myofibrils as judged by the staining pattern of actin and α-actinin ( Fig. 8 ). 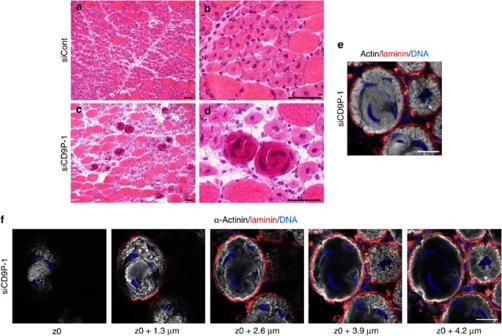Figure 8: Muscle regeneration after grafting of control or CD9P-1-silenced myoblasts. Primary myoblasts were transfected with a siRNA oligonucleotide targeting CD9P-1 (siCD9P-1) or with a control siRNA (siCont) and were grafted into regenerating TA 24 h after a cardiotoxin injury. (a–d) Representative haematoxylin/eosin-stained cross-sections of muscles grafted with control myoblasts (a,b) or CD9P-1-silenced myoblasts (c,d) 4 days after grafting. Scale bar, 50 μm. (e) Three-dimensional projections from 1.3 μm confocal microscopy z-stack of cryosections of TA grafted with CD9P-1-silenced myoblasts stained with 4',6-diamidino-2-phenylindole (DAPI; blue), an anti-laminin antibody (red) and phalloidin to reveal actin (grey). (f) Three-dimensional projections from 1.3 μm successive z-stacks of the same muscle cryosection as inestained with DAPI (blue), an anti-laminin antibody (red) and an anti-α-actinin antibody (grey). Scale bar, 20 μm. (* indicates a normal myoblast). The results are representative of two different silencing experiments, where five mice were grafted with myoblasts treated with a control siRNA in the left TA and with CD9P-1-silenced myoblasts in the right TA. Figure 8: Muscle regeneration after grafting of control or CD9P-1-silenced myoblasts. Primary myoblasts were transfected with a siRNA oligonucleotide targeting CD9P-1 (siCD9P-1) or with a control siRNA (siCont) and were grafted into regenerating TA 24 h after a cardiotoxin injury. ( a – d ) Representative haematoxylin/eosin-stained cross-sections of muscles grafted with control myoblasts ( a , b ) or CD9P-1-silenced myoblasts ( c , d ) 4 days after grafting. Scale bar, 50 μm. ( e ) Three-dimensional projections from 1.3 μm confocal microscopy z-stack of cryosections of TA grafted with CD9P-1-silenced myoblasts stained with 4',6-diamidino-2-phenylindole (DAPI; blue), an anti-laminin antibody (red) and phalloidin to reveal actin (grey). ( f ) Three-dimensional projections from 1.3 μm successive z-stacks of the same muscle cryosection as in e stained with DAPI (blue), an anti-laminin antibody (red) and an anti-α-actinin antibody (grey). Scale bar, 20 μm. (* indicates a normal myoblast). The results are representative of two different silencing experiments, where five mice were grafted with myoblasts treated with a control siRNA in the left TA and with CD9P-1-silenced myoblasts in the right TA. Full size image The skeletal muscle has a remarkable ability to respond to injury by activating a well-orchestrated regenerative response that perfectly restores tissue architecture. The mechanisms underlying the ad integrum restitution of the muscle have remained largely unknown. Our study suggests that the adequate repair of the muscle relies at least in part on a tight control of the fusion ability of myogenic cells, especially myofibres. This conclusion is based on the demonstration that in the absence of the tetraspanins CD9 and CD81, or after silencing their major molecular partner CD9P-1; (a) muscle regeneration is abnormal and characterized by a loss of the normal architecture, and (b) myotubes fuse one to another with a high frequency in vitro , in contrast to control myotubes. The fusion between myotubes in vitro has previously been reported [31] , [32] , and it has also been suggested that some myofibres could fuse one to another in vivo during regeneration [33] . In our conditions, the fusion of two normal myotubes in vitro was a rare event as shown by videomicroscopy. In contrast, in the absence of both CD9 and CD81, or in the absence of CD9P-1, most myotubes fused to other myotubes, leading to the formation of large branched syncytia in vitro . These data strongly suggest the existence of a mechanism preventing the fusion between myotubes, in which these three molecules have a central role. Several data indicate that the abnormal muscle regeneration observed in the absence of CD9 and CD81, or CD9P-1 is at least in part a consequence of dysregulated fusion. First, 4 days after notexin injection, the regenerating muscles of CD9/CD81 null mice display myoblasts with more than three nuclei, in contrast to WT animals. Second, the giant dystrophic structures observed in the absence of these molecules display a number of features suggesting that they result from the abnormal fusion of myofibres. These features include the existence of myofibres with two or three parallel chains of nuclei, apparent merging of two myofibres, and the presence of bundles of myofibrils that are either misaligned or are in different orientations. We therefore conclude that CD9, CD81 and CD9P-1 act as negative regulators of myofibre fusion during the regeneration process, thereby having a major role in maintaining the muscular architecture during this process. Importantly, the dystrophic structures formed during the regeneration of CD9 and CD81 null mice show similarities with abnormal myofibres observed in several myopathies. In particular, the presence in myofibres of actin bundles having different orientations is reminiscent of ring fibres classically associated with late stages of myotonic dystrophies [34] , [35] . It would be interesting to determine whether these abnormal fibres are the result of a defective control of fusion, and to evaluate the function of CD9, CD81 and CD9P-1 in these pathologies. Based on the commonly proposed function of tetraspanins, we hypothesize that CD9 and CD81 might negatively regulate the function of one or several players of myotube fusion through membrane compartmentalization. Our results point to the key role of one of their partners, CD9P-1. The fact that the hyperfusion phenotype is obtained faster on CD9P-1 silencing than in the absence of CD9 and CD81 is consistent with the idea that CD9 and CD81 may function through the regulation of CD9P-1. The function of CD9P-1 is unknown. It was originally described as a protein copurifying with a prostaglandin F2α-binding protein, and was subsequently suggested to negatively modulate the binding of PGF2α on its receptor [36] , [37] . Interestingly, PGF2α was shown to stimulate myoblast fusion [38] . However, the increased fusion observed after CD9P-1 silencing is not due to an increased stimulation of the PGF2α receptor as it is not blocked by inhibition of this receptor ( Supplementary Fig. S4d ). The mTOR pathway was also shown to be required for secondary myoblast/myotube fusion [39] , but was found to be dispensable for the increased myotube/myotube fusion observed on CD9P-1 silencing ( Supplementary Fig. S4e,f ). The recent demonstration that CD9P-1, CD9 and CD81 associate with the γ-secretase complex [40] raised the hypothesis that these molecules could increase the fusion by regulating the Notch pathway, which has a key role in the balance between self-renewal of satellite cells and their engagement towards differentiation [41] . Indeed, γ-secretase-mediated cleavage of Notch is an essential step of this pathway [42] . Inhibition of Notch activity by overexpression of Numb, an antagonist of Notch, or using γ-secretase inhibitor DAPT, was shown to enhance the size of myotubes in vitro by increasing the recruitment of fusing-competent cells [43] . However, the effect of depletion of CD9P-1 is unlikely to be a consequence of altered Notch signalling as we observed no significant change in the expression of Notch targets, hes-1 and hey-1 ( Supplementary Fig. S4g ), that have been demonstrated to be under the control of Notch in adult myogenic progenitors [44] . The precise mechanisms through which CD9P-1 regulates muscle cells fusion will require further investigations. The fusion of myoblasts isolated from CD9 or CD81 null mice was normal while that of CD9/CD81 null mice was greatly enhanced. In vivo , the deletion of only one of these two tetraspanins was sufficient to alter the regeneration process. However the absence of both molecules accelerated the appearance of dystrophic structures. Altogether, these results indicate that while CD9 and CD81 have a similar role during muscle regeneration, they cannot completely compensate for each other during this process. Similar conclusions were reached in other fusion processes: the fertility of CD81 null mice is reduced, but not as much as that of CD9 null mice, and the absence of CD81 in addition to that of CD9 completely abolishes the ability of the egg to fuse with sperm [12] , [13] . In addition, in the absence of either CD9 or CD81 alveolar macrophages had an increased ability to form multinuclear giant cells both in vitro and in vivo , in response to Propionibacterium acnes. However, mice spontaneously developed multinuclear giant cells in the lung only in the absence of both tetraspanins [15] . The similar roles of CD9 and CD81 in several fusion processes are probably linked to their relatively high degree of identity as compared with other tetraspanins, and to their ability to directly associate with the same partner proteins, including CD9P-1 and EWI-2, another protein of unknown function related to CD9P-1 (refs 19 , 20 , 21 , 22 ). It is not known why CD9 and CD81 are either positive or negative regulators of cell fusion depending on the cellular system. This may depend on the nature of the molecules they associate with, or the balance of different associated molecules. In this regard, the expression of EWI-2 is strongly diminished in CD9 null oocytes [45] , which led to the suggestion that the reduced ability of the eggs to fuse in the absence of CD9 could be due to the decreased expression of this molecule. However, a recent report showed that mice lacking EWI-2 had a normal fertility [46] . Of note, EWI-2, in contrast to CD9P-1, did not influence myoblast fusion in this study. In conclusion, this study unveils a mechanism that prevents inappropriate fusion of myogenic cells and that is essential for adequate muscle regeneration. It shows for the first time that a role of tetraspanins in a cell–cell fusion process can be recapitulated by one of their associated proteins, and unravels new role for CD9P-1/EWI-F. Further work should be done to determine how these molecules regulate the fusion process, and their contribution in various pathological muscular conditions where dystrophic myofibres are observed, especially in myotonic dystrophy. Ethical All mice received food and water ad libitum . Before manipulations mice were anaesthetized with an intraperitoneal injection of 0.1 ml per 10 g mouse body weight of a solution containing 1 mg ml −1 xylazine (Rompun 2%, Bayer, Leverkusen, Germany) and 10 mg ml −1 ketamine (Imalgène 1000, Merial, Lyon, France) per mouse. This study was conducted in accordance with the European Communities Council (Directive 2010/63/EU) (ref. 47 ). Mice strains All experiments were conducted with 6- to 8-week-old animals. WT C57BL/6 mice used for tetraspanins expression analysis were obtained from Janvier (Le Genest Saint Isle, France). Tg:Pax7-nGFP mice were described previously [28] . The expression of nGFP corresponds with that of the endogenous Pax7 gene in the embryo and in the adult and labels all satellite cells. C57BL/6 CD81 −/− and CD9 −/− were obtained from the crossing of heterozygotes. The animals were genotyped as previously described [12] , [48] . Double knockout CD9 −/− ::CD81 −/− mice were obtained by successive crossings of the two strains. Muscle injury and tissue preparation For muscle injury, 10 μl of the phospholipase A2 notexin (12.5 μM in PBS, Latoxan, France) were injected intramuscularly with an Hamilton precision syringe into the TA muscle. At various times after injection (4 days, 12 days and 1 month), muscles were dissected and either snap frozen in nitrogen-chilled isopentane and kept at −80 °C, or fixed using buffered 4% paraformaldehyde for 2 h before cryopreservation in 40% sucrose overnight at 4 °C (for Tg:Pax7-nGFP mice), or embedded with the Leica Historesin Embedding kit (Leica Microsystems, Germany) (for analyses in longitudinal section) before sectioning (7, 14 or 1 μm, respectively), haematoxylin and eosin stainings and immunohistochemistry. Microscopic examination was performed with a Nikon 50i microscope with a numeric acquisition system and Nikon NisD software. Grafting experiment Primary myoblasts were transfected with a control siRNA or a siRNA targeting CD9P-1 (see RNA interference section) 1 day after their isolation. Cells (80,000) were grafted by direct intramuscular injection into cardiotoxin-injured regenerating TA (24 h post injury) of C57Bl/6 mice. Primary muscle cell culture Primary myoblasts were isolated from TA muscles of 6-week-old mice by enzymatic digestion as described [49] . All functional experiments were performed with cells isolated from three animals for each genotype. Myoblasts were grown in growth media (Ham’s F10 (PAA), 20% fetal bovine serum, 5 ng ml −1 bFGF (Invitrogen), 100 U ml −1 penicillin G, 100 μg ml −1 streptomycin and neomycin 100 μg ml −1 ) on collagen-coated dishes. For differentiation, myoblasts were plated at 10 5 per well of collagen-coated 24-well dishes and differentiation was induced by switching the growth medium to differentiation medium (DM: DMEM containing 5% horse serum) for different times, the day of the induction is referenced as D0. RNA interference RNA interference was performed using Lipofectamine RNAiMAX reagent (Invitrogen) according to the manufacturer recommendations. The cells were transfected 1 day before and 1 day after the induction of differentiation. All siRNA including the siRNA oligonucleotide control were synthesized by Eurogentec except siCD9P-1_2, which is a stealth siRNA from Invitrogen. They targeted CD81 (5′-GCACCAAATGCATCAAATA-3′), CD9 (5′-GAGCATCTTCGAGCAAGAG-3′), CD9P-1 (siCD9P-1_1: 5′-CATTTGAGATGACTTGCAA-3′ and siCD9P-1_2: 5′-GACACATTCAATTTCCGGATCCAAA-3′) or EWI-2 (5′-GTTCTCCTATGCTGTCTTT-3′). Inhibitor treatments In experiments using inhibitors, vehicle (DMSO: dimethylsulphoxide diluted in DM), AL8810 (10 −6 M) (Cayman), or rapamycin (50 nM) (R&D Systems) were added to DM at D0 and replenished at 24 h for a total treatment of 48 h. When necessary, the cells were fixed and stained with May Grundwald Giemsa and counted. Ten fields of each cell types were photographed at × 10 magnification and the distribution of myotubes according to their nuclei content (1–4; 5–10; 10–30 and more than 30) was determined. Time-lapse imaging Time-lapse Videomicroscopy was performed using an Axiovert 200 inverted microscope (Zeiss, Oberkochen, Germany) equipped with a temperature and CO 2 -controlled chamber. Images were acquired at 10 or 15 min intervals with a Coolsnap HQ camera (Roper Scientific) driven by the Metamorph software (Roper Scientific). Movies were exported and converted into a AVI file displaying images at the speed of 15 frames s −1 . Quantitative reverse transcription–PCR For quantitative reverse transcription–PCR, total RNA fraction was isolated from myoblasts transfected with siRNA control or targeting CD9P-1 after 48 h in DM using Trizol according to the manufacturer’s instructions. Subsequently, cDNA was synthesized from 1 μg of total RNA from each sample using 200 U of SuperScript III Reverse Transcriptase (Invitrogen) primed with random hexamer (Promega). Quantitative real-time polymerase chain reactions (QPCRs) were then carried out in a final volume of 25 μl containing 2 × Brillant II SYBR Green QPCR Master Mix from Agilent, 0.4 μM each forward and reverse primers and 62.5 μg of cDNA. Quantification was performed with the Mx3005P QPCR Systems and MxPro software from Agilent. For each cDNA sample, triplicates were analysed and data normalized to cyclofilin A expression according to the Δ C t method. The primers used for the study are as follows: Hes-1 Forward primer (5′–3′) GAAAGATAGCTCCCGGCATT, reverse primer (5′–3′) GTCACCTCGTTCATGCACTC; Hey-1 Forward primer (5′–3′) GCGCGGACGAGAATGGAAA, reverse primer (5′–3′) TCAGGTGATCCACAGTCATCTG, Cyclofilin A Forward primer (5′–3′) GTCAACCCCACCGTGTTCTT, reverse primer (5′–3′) ACAAGGTCCCAAAGACAGCAG. Antibodies The anti-mouse CD9 (4.1F12) and CD81 monoclonal antibodies (MT81) have been described elsewhere [50] . Two antibodies for CD9P-1 were used: monoclonal antibody 8G1 described in [25] for immunoprecipitation and a sheep polyclonal anti-mouse FPRP from R&D Systems for western blot, FACS analysis and immunohistochemistry (IHC) (10 μg ml −1 ). A goat polyclonal anti-mEWI-2 (10 μg ml −1 ) was purchased from R&D Systems and an anti-mouse α5 integrin mAb MFR5 (10 μg ml −1 ) from BD Pharmingen (Le Pont de Claix, France). The anti-M-cadherin mAb (12G4, 1/20) is from Calbiochem. The monoclonal antibody to Troponin T (JLT-12, 1/500), Myosin Heavy Chain (My-32, 1/1,000), α-actinin (EA-53, 1/5,000) and β-tubulin (tub 2.1, 1/3,000) and the rabbit polyclonal anti-mouse Laminin-2 are from Sigma-Aldrich (Saint-Louis, MO) (1/500). The anti-embryonic Myosin Heavy chain (F1.652, hybridoma supernatant, 1/100) is from the Developmental Studies Hybridoma Bank (DSHB, University of Iowa). Alexa Fluor 488 anti-mouse CD31 (1/500) is from Biolegend. FACS analysis Primary myoblasts were detached at different times of differentiation using a non-enzymic solution, washed and stained with saturating concentrations of primary monoclonal antibody. After washing three times with PBS containing 0.2% BSA, they were incubated with 10 μg ml −1 fluorescein isothiocyanate-labelled secondary antibody. After washing, cells were fixed with 1% formaldehyde in PBS. All incubations were performed for 30 min at 4 °C. Analysis of cell surface staining was performed using a FACSCAN flow cytometer (BD Biosciences). Immunofluorescence microscopy and immunohistochemistry Primary myoblasts were plated on coverslips coated with collagen and induced to differentiate. They were gently rinsed in PBS and fixed for 15 min in 4% paraformaldehyde/PBS at room temperature. The fixed cells were treated for 10 min with 50 mM NH 4 Cl in PBS, washed in PBS and incubated in PBS containing 2% BSA and 10% heat-inactivated goat serum (blocking buffer, BB). Cells were incubated 1 h with the primary antibody diluted in BB, washed three times in BB and incubated with the corresponding secondary anti-rabbit and anti-rat antibodies conjugated to Alexa 488 or Alexa 568 (Molecular Probes/Invitrogen) diluted in BB for 45 min. Coverslips were washed twice with BB and in PBS and then mounted in Mowiol/DABCO (1,4-diazabicyclo[2.2.2]octane) medium. For immunohistochemistry, serial sections of frozen mouse muscle were fixed for 20 min in acetone at −20 °C, dried and stained as above. Actin was labelled by 5 μg ml −1 of phalloidin tetramathylrhodamine isothiocyanate (Sigma-Aldrich) for 15 min. All immunofluorescent stainings were examined with a Leica DMR fluorescence microscope or a TCS SP5 confocal microscope (Leica, Wetzlar, Germany). To produce three-dimensional projection images we captured frames every 0.13 μm to create the z-axis series, which were then combined and processed using the ImageJ sofware. Immunoprecipitation and western blot For direct western blot, cells were lysed at 4 °C in RIPA lysis buffer containing 10 mM Tris, pH 7.4, 150 mM NaCl, 0.02% NaN 3 , protease inhibitors, and 1% NP-40, 0.5% deoxycholic acid and 0.1% SDS. Cell extracts were centrifugated at 10,000 r.p.m. for 15 min. For immunoprecipitations, myoblasts were surface labelled or not with EZ-link-Sulfo-NHS-LC-biotin (Pierce, Rockford, IL, USA) as described previously before lysis in 1% Brij97 at 4 °C and immunoprecipitations using Protein G–Sepharose beads (Amersham Biosciences, Rainham, Essex, UK), as previously described [19] , [20] . After protein separation by SDS–PAGE and transfer to a nitrocellulose membrane, the membranes were incubated with indicated primary antibody and the expression of each protein was revealed with appropriate secondary antibodies labelled with Alexa Fluor 680 (Invitrogen) or IrDye800 (LI-COR). Biotin-labelled surface proteins were revealed using Alexa Fluor 800-labelled streptavidin (Invitrogen). The data were acquired using the Odyssey Infrared Imaging System (LI-COR Biosciences). Statistical analysis All statistical analyses were performed using the Mann–Whitney test. How to cite this article: Charrin, S. et al . Normal muscle regeneration requires tight control of muscle cell fusion by tetraspanins CD9 and CD81. Nat. Commun. 4:1674 doi: 10.1038/ncomms2675 (2013).